An asymmetric allelic interaction drives allele transmission bias in interspecific rice hybrids Hybrid sterility (HS) between Oryza sativa (Asian rice) and O . glaberrima (African rice) is mainly controlled by the S1 locus. However, our limited understanding of the HS mechanism hampers utilization of the strong interspecific heterosis. Here, we show that three closely linked genes ( S1A4 , S1TPR , and S1A6 ) in the African S1 allele ( S1-g ) constitute a killer-protector system that eliminates gametes carrying the Asian allele ( S1-s ). In Asian–African rice hybrids ( S1-gS1-s ), the S1TPR-S1A4-S1A6 interaction in sporophytic tissues generates an abortion signal to male and female gametes. However, S1TPR can rescue S1-g gametes, while the S1-s gametes selectively abort for lacking S1TPR. Knockout of any of the S1-g genes eliminates the HS. Evolutionary analysis suggests that S1 may have arisen from newly evolved genes, multi-step recombination, and nucleotide variations. Our findings will help to overcome the interspecific reproductive barrier and use Asian–African hybrids for increasing rice production. Hybrid sterility (HS) is a major mechanism of postzygotic reproductive isolation, which can limit reproduction among divergent populations during speciation and thus contribute to the maintenance of species identity [1] , [2] . The classic Bateson–Dobzhansk–Muller (BDM) model [3] attributes postzygotic reproductive isolation to an incompatible genetic interaction between divergent alleles of at least two loci [4] , [5] , although mounting evidence suggests that HS caused by the interaction of alleles comprising multiple genes at a single locus also fits the BDM model [6] , [7] , [8] , [9] , [10] , [11] , [12] , [13] , [14] , [15] . The HS loci act as selfish genetic elements, which can eliminate the gametes carrying competing alleles, thus gaining a transmission advantage over other alleles, similar to meiotic drive. This can result in distorted segregation and non-Mendelian transmission of the alleles in the progenies [6] , [7] , [8] , [9] , [10] , [11] , [12] , [13] , [14] , [15] . The killer–protector system and killer meiotic driver models have been proposed to explain the biased allele transmission of HS in eukaryotes [14] , [16] . In this model, the killer gene (usually functioning in the sporophyte) produces a detrimental sterility signal that indiscriminately kills all meiotic cells [16] . The protector gene (usually tightly linked to the killer gene) functions in the gamete to eliminate this detrimental effect and rescue the gamete that contains the correct allele of the protector gene. Therefore, gametes carrying the protector gene survive; gametes lacking the protector gene die [16] . The Oryza genus comprises 21 wild species and 2 cultivated species, Asian rice ( O . sativa L., including the subspecies japonica and indica ) and African rice ( O . glaberrima Steud.) [17] , [18] . The broad genetic diversity within Oryza can contribute to heterosis, also known as hybrid vigor, in which the hybrid performs better than its parental inbred lines [19] , [20] . However, HS of different forms (e.g., male sterility, female sterility, and both male and female sterilities) is common between different species and subspecies in the Oryza genus and this HS hinders the ability of plant breeders to use the strong heterosis in the production of high yield, robust hybrid rice. Therefore, understanding the mechanisms of the HS could enable breeding of improved hybrid rice. A number of HS loci have been genetically studied in Oryza [19] , [20] and several HS genes have been cloned from various loci, including the single-locus HS loci Sa , S5 , HSA1 , S7 , S1 , Sc , qSHMS7 , ESA1 , and the two-locus DPL1 / DPL2 , S27 / S28 , and DGS1 / DGS2 pairs [8] , [12] , [14] , [15] , [21] , [22] , [23] , [24] , [25] , [26] , [27] , [28] , [29] . Despite extensive studies of these loci, our understanding of the molecular mechanisms governing HS and its effect on genome evolution remains limited. S1 is a typical single-locus-type HS locus that affects hybrids produced by crossing African and Asian rice [23] , [27] , [30] , [31] , [32] . In these Asian–African rice hybrids, male and female gametes carrying the Asian rice S1 allele ( S1-s ) are selectively aborted, leading to very strong preferential transmission of the African rice S1 allele ( S1-g ), which reaches an allele frequency of ca. 0.95 in F 2 progeny [27] . Recently, we cloned OgTPR1 , the peptidase-encoding causal gene of the HS effect of the S1 locus; another S1 -related gene, SSP , also encoding a peptidase, was later identified by Koide and colleagues [23] . Despite these advances, the molecular mechanism governing the selective abortion and survival of gametes with different alleles in interspecific and intersubspecific hybrids in plants remains poorly understood, and the evolutionary origins of HS loci and their relationship to speciation remain largely unknown. Here, we identify additional HS-related genes at S1 , describe the S1 tripartite gamete killer–protector system, and explore the evolutionary relationship of this complex locus with the allopatric speciation of the related Oryza species. The S1A4 gene is required for S1 HS Our previous study revealed the existence of structural variation between the African rice S1 allele ( S1-g ) and the Asian rice S1 allele ( S1-s ) [27] . We found that OgTPR1 (hereafter named S1TPR ) at S1-g is required for S1 -mediated HS. Moreover, S1-s contains an S1TPR allele, named S1TP , which is a truncated form of S1TPR due to a premature stop codon caused by a single-nucleotide mutation (Fig. 1a ) [27] . According to our sequence analysis, besides S1TPR , the S1-g region contains six African rice-specific putative genes, S1A1 – S1A6 (Fig. 1a ). We determined the expression profiles of these genes in a near-isogenic line carrying S1-g (NIL- g ) and its recurrent parental line RP- s ( japonica rice carrying S1-s ), and their F 1 plants. This showed that S1A2–S1A6 were transcriptionally active in anthers and young panicles (Supplementary Figs. 1a and 2 ). Moreover, S1TPR was expressed at high levels in the microspores (Supplementary Fig. 1b ) Fig. 1 S1A4 - S1TPR - S1A6 constitutes a killer–protector system. a The structures of the African rice allele S1-g ( g ) and Asian rice allele S1-s ( s ). A point (C-to-A) mutation of S1TPR ( TPR ) results in a premature stop codon in S1TP ( TP ). African rice-specific sequences are in green. Six putative genes specific to African rice, S1A1 – S1A6 ( A1 – A6 ), were located in S1-g . Red arrows, CRISPR/Cas9 target sites. b – d The fertility of the transgenic plants of RP- s (the recurrent parent of O . sativa ssp. japonica with ss ) and their hybrids carrying different combinations of the transgenes TPR t ( T ) and linked A4 – A6 t ( 46 ). The T 0 plants carrying one ( b ) or two ( c ) transgenes were fully fertile (FF, ~95% fertility), as observed in their pollen (top) and spikelets (bottom); however, the co-existence of the three transgenes (all in hemizygous state; ‘–’ denotes absence of the T-DNA/transgene in the chromosome site) induced semi-sterility (SS, 45~55% sterility) of the pollen and spikelets (green spikelets are sterile). d Bars, 50 μm for pollen and 5 cm for panicles. e The segregation of the A4–A6 t and TPR t transgenes in the T 1 family, and the segregation of the A4–A6 t in F 2 population derived from A4 – A6 t (homozygote) × TPR t (homozygote) fit the 1:2:1 ratio, but the segregation of the TPR t transgene in this F 2 population was significantly distorted (*** P < 0.001 in the Χ 2 test) from the ratio. f A deduced model for the segregation behavior of the transgenes in the F 2 progeny derived from A4 – A6 t × TPR t . The F 1 male and female gametes containing T are fertile, and those lacking T are generally sterile. The color codes are consistent with the genotype of the individuals in the F 2 population. Black represents homozygous TPR t ; dark orange represents homozygous A4 – A6 t ; orange represents hemizygous A4 – A6 t ; light orange represents lacking A4 – A6 t . Source data of ( e ) are provided as a Source Data file Full size image To test whether S1TPR is sufficient to cause gamete abortion, we generated transgenic plants that contained an S1TPR transgene ( S1TPR t ) in the RP- s background. The T 0 plants hemizygous for S1TPR t ( S1TPR t –, where dash indicates absence of the T-DNA/transgene in the chromosome site) had fully fertile pollen and spikelets (Fig. 1b ), indicating that S1TPR is not sufficient to induce HS. These results suggest that S1 HS requires other O . glaberrima -specific S1 component(s) in addition to S1TPR . To investigate whether any of the anther- and panicle-expressed S1 genes ( S1A2 – S1A6 ) are involved in S1 HS, we used CRISPR/Cas9 to individually knock out their functions in NIL- g . All the obtained knockout mutants ( s1a2–s1a6 ) showed normal male and female fertility, which indicates that these genes are not essential for gamete development (Supplementary Fig. 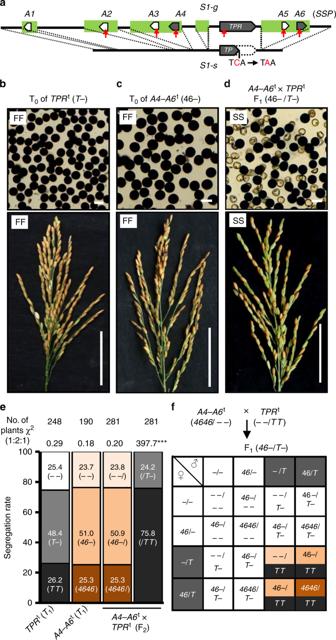Fig. 1 S1A4-S1TPR-S1A6constitutes a killer–protector system.aThe structures of the African rice alleleS1-g(g) and Asian rice alleleS1-s(s). A point (C-to-A) mutation ofS1TPR(TPR) results in a premature stop codon inS1TP(TP). African rice-specific sequences are in green. Six putative genes specific to African rice,S1A1–S1A6(A1–A6), were located inS1-g. Red arrows, CRISPR/Cas9 target sites.b–dThe fertility of the transgenic plants of RP-s(the recurrent parent ofO.sativassp.japonicawithss) and their hybrids carrying different combinations of the transgenesTPRt(T) and linkedA4–A6t(46). The T0plants carrying one (b) or two (c) transgenes were fully fertile (FF, ~95% fertility), as observed in their pollen (top) and spikelets (bottom); however, the co-existence of the three transgenes (all in hemizygous state; ‘–’ denotes absence of the T-DNA/transgene in the chromosome site) induced semi-sterility (SS, 45~55% sterility) of the pollen and spikelets (green spikelets are sterile).dBars, 50 μm for pollen and 5 cm for panicles.eThe segregation of theA4–A6tandTPRttransgenes in the T1family, and the segregation of theA4–A6tin F2population derived fromA4–A6t(homozygote) ×TPRt(homozygote) fit the 1:2:1 ratio, but the segregation of theTPRttransgene in this F2population was significantly distorted (***P< 0.001 in theΧ2test) from the ratio.fA deduced model for the segregation behavior of the transgenes in the F2progeny derived fromA4–A6t×TPRt. The F1male and female gametes containingTare fertile, and those lackingTare generally sterile. The color codes are consistent with the genotype of the individuals in the F2population. Black represents homozygousTPRt; dark orange represents homozygousA4–A6t; orange represents hemizygousA4–A6t; light orange represents lackingA4–A6t. Source data of (e) are provided as a Source Data file 3a and Supplementary Table 1 ). If a specific gene is required for S1 HS, knocking it out in NIL- g should create a neutral allele that does not show HS in crosses with RP- s . When these mutants were crossed with RP- s , the mutant F 1 plants containing the s1a2 , s1a3 , or s1a5 mutant alleles were semi-sterile (ca. 50% sterile pollen grains and spikelets) (Supplementary Fig. 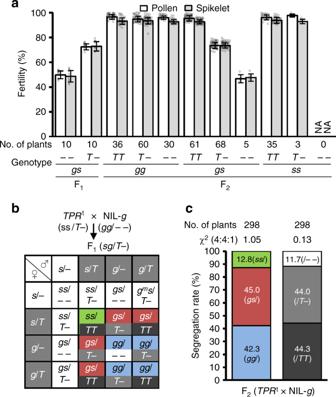Fig. 2 TheS1TPRtrescues the gametes carryingS1-sin hybrids.aPollen and spikelet fertilities of the F1plants derived from the cross between the hemizygousS1TPRt(TPRt,ss/T–) and NIL-g(gg/– –), and various genotypes of the F2segregants. Error bars indicate S.D. NA, not available.bA proposed model for the segregation behavior of the endogenousS1alleles andTPRtin the F2plants derived fromTPRt× NIL-g. The F1male and female gametes containingS1-gand/orTare considered fertile, and those withS1-s(ss/– –) but lackingTare generally sterile. Thus, the expected segregation ratios forgg:gs:ssandTT:T–:– – are 4:4:1. The color codes are consistent with the genotype of the individuals in the F2population. Black represents homozygousTPRt; gray represents hemizygousTPRt; white represents lackingTPRt; green represents homozygousS1-s; red represents heterozygousS1; blue represents free homozygousS1-g.cThe segregation rates of theS1alleles and the transgene (T) in the analyzed F2population fit the expected ratio. Source data of (a,c) are provided as a Source Data file 3b and Supplementary Table 2 ), like the RP- s × NIL- g F 1 plants (see below Fig. 3a ). However, the mutant F 1 plants containing the s1a4 and s1a6 alleles were fully fertile (Supplementary Fig. 3b and Supplementary Table 2 ), suggesting that S1 HS requires S1A4 and S1A6 . This result is consistent with a recent report that SSP , which corresponds to S1A6 , is involved in S1 HS [23] . Moreover, we found that in the s1a4 and s1a6 mutant lines, agronomic traits including plant architecture, grain length, grain width, plant height, panicle length, and grain number per panicle were not significantly different compared to NIL- g , but their 1000-grain weight was slightly heavier than that of NIL- g (Supplementary Fig. 4 ). These results suggest that S1A4 and S1A6 may have a pleiotropic effect on the seed-filling process in addition to their roles in HS. S1A4 - S1TPR - S1A6 constitutes a killer–protector system To understand whether S1A4 , S1TPR , and S1A6 are sufficient to kill gametes, we transformed RP- s with transgenes containing different combinations of these three genes, then looked for sterility and distortion of segregation of the transgenes. If the killing process requires all three genes, gamete abortion would not occur in plants carrying only one or two of these components. Indeed, all the plants transformed with one ( S1TPR t , S1A4 t , or S1A6 t ), or two transgenes (the S1A4–S1A6 t and S1TPR-S1A6 t transgenes carrying two genes, or the pyramided transgenes in the F 1 of S1A4 t × S1TPR t ), all in a hemizygous state, did not show the typical semi-sterile phenotypes of pollen and spikelets (Fig. 1c and Supplementary Fig. 5 ). In contrast, when the three transgenes were pyramided together by a cross between the homozygous S1A4 – S1A6 t and S1TPR t lines, the pollen and spikelets of the transgenic F 1 plants were semi-sterile (Fig. 1d ). Furthermore, abnormal embryo sacs were observed in the F 1 plants of S1A4 – S1A6 t × S1TPR t (Supplementary Fig. 6 ), consistent with previous reports in Asian–African rice hybrids [23] , [31] . These results suggested that these three genes are necessary and sufficient to constitute a gamete-killer system. We further analyzed the segregation of the S1A4 – S1A6 t and S1TPR t transgenes. The segregation of S1TPR t and S1A4 – S1A6 t in their T 1 generations fit the 1:2:1 ratio, consistent with the hypothesis that the HS requires all three components (Fig. 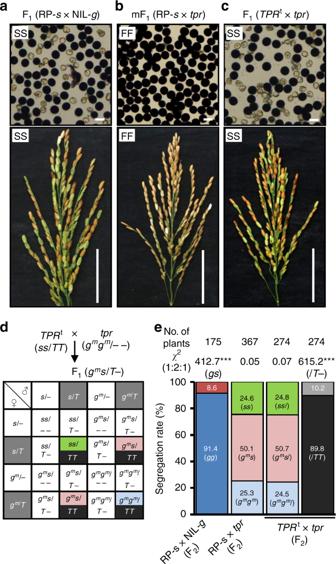Fig. 3 Dual functions ofS1TPRinS1HS.aF1hybrids from crossing RP-swith NIL-gexhibited typical semi-sterile pollen and spikelets.bThe pollen and spikelets of the mutant F1(mF1) plants from crosses between RP-sand the CRISPR-knockout mutants1tpr(tpr) in NIL-g(gmgm) were fully fertile.cThe F1plants from a cross between theS1TPRt(TPRt,ss/TT) andtpr(gmgm) lines exhibited semi-sterile pollen and spikelets. Bars in (a–c) represent 50 μm for pollen and 5 cm for panicles.dA proposed model for the segregation of theS1alleles and transgenes in the F2progeny of theTPRt×tprcross. The F1male and female gametes containing theTallele (gray background) are fertile, and those withoutT(white background) generally abort. The color codes are consistent with the genotype of the individuals in the F2population. Black represents homozygousTPRt; green represents homozygousS1-s; pink represents heterozygous mutatedS1; light blue represents homozygous mutatedS1-gm.eSegregation rates of theS1alleles and transgenes (T) in the F2plants shown in (a–c). ***P<0.001 in theΧ2test. Source data of (e) are provided as a Source Data file 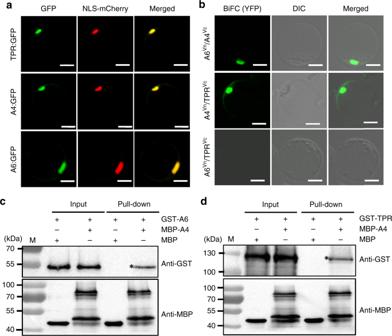Fig. 4 S1TPR-S1A4–S1A6 is a tripartite complex in the nucleus.aS1TPR (TPR, top), S1A4 (A4, middle), and S1A6 (A6, bottom) were fused with GFP and each was co-expressed with the nuclear localization signal marker (NLS-mCherry) in the rice protoplasts. The GFP fluorescence perfectly matched the mCherry fluorescence. Scale bars, 10 μm.bBiFC assays showed that, in the nuclei of rice protoplasts, A4 interacts with A6 and TPR (top and middle), but A6 does not interact with TPR (bottom). Scale bar, 10 μm.c,dPull-down assays confirmed that A4 interacts with A6 (c) and TPR (d) in vitro. “*” indicates the MBP-A4 pull-down proteins (GST-A6 or GST-TPR) detected using the anti-GST antibody. M means 10–180 kDa protein size marker (Thermo Fisher Scientific, CA, USA). Source data of (c,d) are provided as a Source Data file 1e , Supplementary Tables 3 and 4 ). As expected, the F 1 of the S1A4 – S1A6 t × S1TPR t cross (sporophytic genotype S1A4 – S1A6 t –/ S1TPR t –) was semi-sterile. Moreover, the segregation of S1TPR t was severely distorted, with most (75.8%) of the F 2 individuals carrying homozygous S1TPR t and the rest containing hemizygous S1TPR t (Fig. 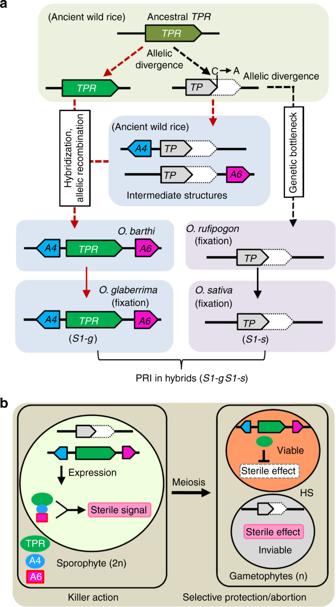Fig. 5 Evolution and mechanism of theS1killer–protector system.aA simplified evolutionary trajectory of theS1alleles inOryza. CurrentS1TPR(TPR) andS1TP(TP) alleles in theOryzagenus might be derived from the ancestralTPRgenes from two independent lineages. In one lineage, the divergedTPalleles passed through a bottleneck and migrated intoO.rufipogon, eventually being fixed asS1-sinO.sativa. In another lineage, the intermediate structures (A4-TPandTP-A6) carrying the new genesS1A4(A4) andS1A6(A6) arose in ancient wild rice, and theA4-TPR-A6three-gene structure were generated inO.barthii, probably by natural hybridization and allelic recombination; this structure further migrated intoO.glaberrimaas the functionalS1-gallele. In hybrids betweenO.glaberrimaandO.sativa, this gamete killer–protector system causes postzygotic reproductive isolation (PRI).bA working model for theS1gamete killer–protector system in African-Asian rice hybrids. In the sporophytic cells (megaspore/microspore mother cells) of the hybrids, the three-protein complex, comprising TPR, A4, and A6, expressed fromS1-gmay produce a sterility-trigging signal. This signal is retained in the post-meiotic male and female gametes and causes the selective abortion of gametes carryingS1-s, whereas TPR in theS1-ggametes eliminates the sterility.S1-gtherefore has a strong transmission advantage in the hybrids and acts as a typical ultra-selfish genetic element 1e and Supplementary Table 5 ). This indicated that the gametophytic genotype is what matters for the transmission advantage of S1TPR t . However, the segregation ratio of S1A4 – S1A6 t in the F 2 progeny of S1A4 – S1A6 t × S1TPR t fit the 1:2:1 ratio, similar to the segregation of S1TPR t and S1A4 – S1A6 t in their T 1 generations (Fig. 1e , Supplementary Tables 3 – 5 ). Since S1A4 – S1A6 t and S1TPR t are not linked, this is consistent with S1TPR t in the gametophyte providing protection from the sterile effect of S1A4 – S1A6 t and S1TPR t in the sporophyte. In contrast to the situation in the native S1-g allele, here the transgenes are unlinked and the distortion of S1TPR t segregation does not affect the normal S1A4 – S1A6 t segregation. Moreover, it is consistent with the effect of S1A4 – S1A6 t and S1TPR t acting in the sporophyte. These observations prompted us to propose a model using a Punnett square to explain the results of this genetic analysis (Fig. 1f ). We reasoned that S1A4 , S1TPR , and S1A6 might act together in the sporophyte to produce a detrimental sterility signal that kills the male and female gametes. However, the S1TPR t transgene alone is capable of protecting the corresponding gametes (with or without S1A4 – S1A6 t ) from the sterility, thereby rescuing the gametes harboring S1TPR t and leading to severely distorted segregation favoring S1TPR t in the F 2 progeny but not affecting segregation of the unlinked S1A4 – S1A6 t . S1TPR is required for killer and protector function If S1TPR in the gamete is sufficient to provide the protector function at the S1 locus, gametes containing the S1-s allele should be partially rescued by the S1TPR transgene. To test this, we crossed the hemizygous S1TPR t line with NIL- g to produce F 1 hybrids ( S1-gS1-s / S1TPR t –) that contain the S1-g allele in the sporophytic tissue (and thus should activate HS), but will segregate the S1TPR t transgene in the gametes. Indeed, the F 1 and F 2 plants that are heterozygous for S1 but lack the S1TPR t transgene were semi-sterile (~50%). By contrast, the fertilities of the pollen and spikelets of the F 1 and F 2 plants that are heterozygous for S1 and carry the S1TPR t transgene in a hemizygous condition increased to ~75%. Moreover, the S1 -heterozygotes with homozygous S1TPR t were fully fertile (Fig. 2a and Supplementary Table 6 ), indicating that the S1TPR t allows transmission of the S1-s allele carrying this transgene. The F 2 plants homozygous for S1 ( S1-sS1-s or S1-gS1-g ) were fully fertile regardless of whether they contained S1TPR t or not (Fig. 2a and Supplementary Table 6 ). This suggests that S1TPR t indeed rescued the gametes containing S1-s in a gametophytic manner. Fig. 2 The S1TPR t rescues the gametes carrying S1-s in hybrids. a Pollen and spikelet fertilities of the F 1 plants derived from the cross between the hemizygous S1TPR t ( TPR t , ss / T –) and NIL- g ( gg /– –), and various genotypes of the F 2 segregants. Error bars indicate S.D. NA, not available. b A proposed model for the segregation behavior of the endogenous S1 alleles and TPR t in the F 2 plants derived from TPR t × NIL- g . The F 1 male and female gametes containing S1-g and/or T are considered fertile, and those with S1-s ( ss /– –) but lacking T are generally sterile. Thus, the expected segregation ratios for gg : gs : ss and TT : T –:– – are 4:4:1. The color codes are consistent with the genotype of the individuals in the F 2 population. Black represents homozygous TPR t ; gray represents hemizygous TPR t ; white represents lacking TPR t ; green represents homozygous S1-s ; red represents heterozygous S1 ; blue represents free homozygous S1-g . c The segregation rates of the S1 alleles and the transgene ( T ) in the analyzed F 2 population fit the expected ratio. Source data of ( a , c ) are provided as a Source Data file Full size image Based on these findings and our hypothesis, we proposed that in the F 1 plants ( S1-gS1-s / S1TPR t –) of S1TPR t × NIL- g , the S1-g allele produced a sterility signal in the sporophytic cells. However, all the S1-g- containing gametes survive due to the presence of the endogenous S1TPR , and the S1-s- containing gametes are aborted unless they carried the S1TPR t transgene. The segregation ratios for the genotypes of S1 ( S1-gS1-g : S1-gS1-s : S1-sS1-s ) and S1TPR t ( S1TPR t S1TPR t : S1TPR t –:– –) were therefore predicted to be 4:4:1 in the F 2 population (Fig. 2b ). Indeed, this segregation ratio perfectly fit the ratio from genetic analysis of the S1TPR t × NIL- g F 2 population (Fig. 2c and Supplementary Table 6 ). To further verify that S1TPR also participates in the killing process, we crossed the homozygous S1TPR t plants with the s1tpr mutant (the function of S1TPR was completely knocked out, resulting in homozygous mutated S1-g m ) [27] . We reasoned that if the S1TPR t transgene can function together with the endogenous S1A4 and S1A6 (still present at the S1-g m allele) genes to kill the gametes, gamete abortion would be observed in the resultant F 1 hybrids. As expected, the F 1 plants exhibited semi-sterile pollen and spikelets, like those of RP- s × NIL- g (Fig. 3a–c ). Since S1TPR makes up part of the killer system, and has another role in the protection of S1TPR -containing gametes, we therefore hypothesized a segregation model, in which the hybrids ( S1-g m S1-s / S1TPR t –) produce a detrimental sterility signal (in a sporophytic manner) to kill the gametes carrying S1-s or S1-g m , but the S1TPR t -containing gametes survive (Fig. 3d ). As expected, in the F 2 population of the S1TPR t × s1tpr cross the segregation ratio of the S1 genotypes ( S1-g m S1-g m : S1-g m S1-s : S1-sS1-s ) fit the 1:2:1 ratio, and the S1TPR t genotypes had a significantly distorted segregation ratio (Fig. 3e and Supplementary Table 7 ). These results also suggested that the abortion of the S1-s or S1-g m -containing gametes in the hybrids is independent of the S1TP gene at S1-s or other gametophytic responder genes. Fig. 3 Dual functions of S1TPR in S1 HS. a F 1 hybrids from crossing RP- s with NIL- g exhibited typical semi-sterile pollen and spikelets. b The pollen and spikelets of the mutant F 1 (mF 1 ) plants from crosses between RP- s and the CRISPR-knockout mutant s1tpr ( tpr ) in NIL- g ( g m g m ) were fully fertile. c The F 1 plants from a cross between the S1TPR t ( TPR t , ss / TT ) and tpr ( g m g m ) lines exhibited semi-sterile pollen and spikelets. Bars in ( a – c ) represent 50 μm for pollen and 5 cm for panicles. d A proposed model for the segregation of the S1 alleles and transgenes in the F 2 progeny of the TPR t × tpr cross. The F 1 male and female gametes containing the T allele (gray background) are fertile, and those without T (white background) generally abort. The color codes are consistent with the genotype of the individuals in the F 2 population. Black represents homozygous TPR t ; green represents homozygous S1-s ; pink represents heterozygous mutated S1 ; light blue represents homozygous mutated S1-g m . e Segregation rates of the S1 alleles and transgenes ( T ) in the F 2 plants shown in ( a – c ). *** P < 0.001 in the Χ 2 test. Source data of ( e ) are provided as a Source Data file Full size image S1A6-S1A4-S1TPR is a tripartite complex in the nucleus In this gamete killer–protector system, S1A6 encodes a smaller peptidase with similar features to the S1TPR peptidase [23] , [27] , and S1A4 encodes an uncharacterized protein of 261 amino acids without any putative conserved domains (Supplementary Fig. 7 ). To study the subcellular localization of these proteins, S1A4 , S1A6 , and S1TPR were fused with the GFP gene sequence, respectively, and expressed in rice protoplasts. All these proteins localized in the nucleus (Fig. 4a ), suggesting that they may interact with each other in the nucleus. Consistent with this, bimolecular fluorescence complementation (BiFC) and pull-down assays indicated that S1A4 interacted with S1A6 and S1TPR respectively in the nucleus, but S1TPR did not interact with S1A6 directly (Fig. 4b–d ). Fig. 4 S1TPR-S1A4–S1A6 is a tripartite complex in the nucleus. a S1TPR (TPR, top), S1A4 (A4, middle), and S1A6 (A6, bottom) were fused with GFP and each was co-expressed with the nuclear localization signal marker (NLS-mCherry) in the rice protoplasts. The GFP fluorescence perfectly matched the mCherry fluorescence. Scale bars, 10 μm. b BiFC assays showed that, in the nuclei of rice protoplasts, A4 interacts with A6 and TPR (top and middle), but A6 does not interact with TPR (bottom). Scale bar, 10 μm. c , d Pull-down assays confirmed that A4 interacts with A6 ( c ) and TPR ( d ) in vitro. “*” indicates the MBP-A4 pull-down proteins (GST-A6 or GST-TPR) detected using the anti-GST antibody. M means 10–180 kDa protein size marker (Thermo Fisher Scientific, CA, USA). Source data of ( c , d ) are provided as a Source Data file Full size image Possible biochemical effect of the S1 -HS system Given that the S1 HS factors interact in the nucleus, we next examined their effects on the transcriptome. To determine which biochemical processes cause gamete abortion and to explore the possible mechanisms by which this occurs, we sequenced the transcriptomes of anthers (at the microspore mother cell stage to meiosis stage) from RP- s , NIL- g , and their F 1 hybrids. We identified 250 commonly upregulated genes and 74 commonly downregulated genes in the NIL- g and F 1 plants relative to their levels in RP- s (Supplementary Fig. 8a ). These genes were then analyzed using the KEGG pathway database ( http://www.genome.jp/kegg/ ), revealing that the expressions levels of genes involved in photosynthesis and the degradation of valine, leucine, and isoleucine (branched-chain amino acids, BCAAs) were significantly upregulated in the NIL- g and F 1 plants versus the RP- s plants (Supplementary Figs. 8b and 9 ). However, the analysis did not identify any significantly enriched pathway among the downregulated genes. The expression profiles of these differentially expressed genes involved in photosynthesis and BCAA degradation were further confirmed using qRT-PCR (Supplementary Fig. 10 ). These results hinted that photosynthesis and BCAA may be associated with gamete development. Evolutionary origin of the S1 gamete killer–protector system According to the BDM model, hybrid incompatibility is caused by a detrimental interaction between the divergent alleles of two independent lineages, which may have been derived from a recent common ancestor [4] . To trace the evolution of the S1 locus, we first used the S1TPR , S1TP , S1A4 , and S1A6 nucleotide coding sequences to perform a BLAST search for putative orthologs in the Poaceae sequences using the GenBank database ( https://www.ncbi.nlm.nih.gov/ ), and constructed a phylogenetic tree of the candidates. We found that the nucleotide coding sequences of S1TPR , but not S1A4 and S1A6 , were significantly similar to rice in the genomes of Zea mays , Sorghum bicolor , Brachypodium distachyon , Hordeum vulgare , Aegilops tauschii , Triticum aestivum , and Setaria italica (Supplementary Fig. 11 ). Notably, the orthologous gene (LOC101754700) in S . italica has the highest nucleotide identity (ca. 82%) with S1TPR and S1TP . Thus, the S1TPR ortholog in S . italic is used as one of the appropriate outgroup references for analyzing the divergence of S1TPR and S1TP . To further confirm the point of divergence in the S1 locus of Oryza , we identified the S1TPR , S1TP , S1A4 , and S1A6 sequences in the AA genome species of Oryza ( O . meridionalis , O . longsistaminata , O . barthii , O . rufipogon , O . glaberrima , and O . sativa ) and several non-AA genome species, including O . officinalis (CC genome), O . rhizomatis (CC genome), O . eichingeri (CC genome), and O . minuta (BBCC genome), which are all closely related to the AA genome Oryza species based on molecular evidence [33] . These non-AA genome species were also used as outgroups in the divergent analysis of the genes. We found that only S1TPR and/or S1TP , but not S1A4 and S1A6 , were present in these outgroup species, indicating that S1A4 and S1A6 likely newly evolved in the Oryza species with AA genomes (Supplementary Fig. 12 and Supplementary Data 1 ). Since seven single-nucleotide polymorphisms (SNPs, sites 1–7) are present between the S1TPR and S1TP coding sequences (Supplementary Fig. 12 ) [27] , we further analyzed the patterns of these seven SNPs in 443 accessions of the AA-genome Oryza species and some other outgroup species (including S . italica ) to trace the sequence divergence of the S1TPR and S1TP genes in these species. An S1TPR -type allele (Allele 1) was detected in S . italica , O . officinalis , O . minuta , O . longsistaminata , and O . meridionalis (Supplementary Fig. 12 and Supplementary Data 1 ), thus likely representing the primitive form of S1TPR . Notably, the nucleotides at SNP site 7 (C to A variation causing the premature stop codon in S1TP ) were polymorphic not only among the AA genome species, but also among the analyzed CC genome species. In contrast, the polymorphisms of the SNP sites 1–6 were present only in AA genome species (Supplementary Fig. 12 and Supplementary Data 1 ), suggesting that SNP 7 in S1TPR and S1TP arose early in the evolution of the Oryza genus and that various alleles co-existed in the primitive Oryza gene pool. On the basis of these detected SNP patterns, we identified at least fifteen S1TP alleles (Alleles 1–1 to 1–15) that contained variations at the SNP sites 1, 3, 4, 6, and 7 in AA-genome Oryza species, including O . longistaminata , O . meridionalis , O . rufipogon , and O . sativa . All O . rufipogon accessions (68) and all O . sativa accessions (116) carried the one-gene S1 structure containing S1TP (haplotype). Furthermore, we found four S1TPR alleles (Alleles 2-1 to 2–4) that carried variations at the SNP sites 2 and 5 in O . barthii and O . glaberrima (Supplementary Fig. 12 ). The non-overlapping natural variations in the S1TPR and S1TP alleles between O . glaberrima and O . sativa suggested that at least two independent lineages evolved from the common ancestral lineage carrying the ancestral S1TPR gene (Fig. 5a , Supplementary Figs. 12 and 13 ). In one lineage, the resultant S1TP variants (Alleles 1-1 to 1–16) passed a bottleneck and some (Alleles 1–3 to 1–8) were transmitted into O . rufipogon , resulting in the eventual fixing of two (Alleles 1–3 and 1–8) as the current S1 - s in O . sativa ; this allele is present in all populations of O . sativa (Fig. 5a , Supplementary Figs. 12 and 13 ). By contrast, S1-g likely evolved in another lineage (Fig. 5a , Supplementary Figs. 12 and 13 ). Given that S1A4 and S1A6 are absent in the CC and BBCC genomes of other Oryza species, we speculated that the S1A4 - S1TPR / S1TP-S1A6 alleles might newly evolve in the AA-genome Oryza species. Consistent with this hypothesis, three types of S1TP -containing structures with the genes S1A4 and/or S1A6 , inserted upstream and downstream of S1TP , respectively, were identified in O . meridionalis (Fig. 5a , Supplementary Figs. 12 and 13 ). Seven accessions had the S1A4-S1TP structure (Alleles 1–9 to 1–11), five accessions had the S1TP-S1A6 structure (Alleles 1–12 and 1–13), and two accessions had the S1A4-S1TP-S1A6 structure (Alleles 1–14 and 1–15) (Fig. 5a , Supplementary Figs. 12 and 13 ). Similarly, three types of S1TPR -containing structures with S1A4 and/or S1A6 (Alleles 2–2 to 2–4) were identified in O . barthii , the wild progenitor of O . glaberrima (Fig. 5a , Supplementary Figs. 12 and 13 ): 10 accessions had the S1A4-S1TPR structure, one accession had the S1TPR-S1A6 structure, and 52 accessions had the three-gene structure S1A4-S1TPR-S1A6 (Fig. 5a , Supplementary Figs. 12 and 13 ). Fig. 5 Evolution and mechanism of the S1 killer–protector system. a A simplified evolutionary trajectory of the S1 alleles in Oryza . Current S1TPR ( TPR ) and S1TP ( TP ) alleles in the Oryza genus might be derived from the ancestral TPR genes from two independent lineages. In one lineage, the diverged TP alleles passed through a bottleneck and migrated into O . rufipogon , eventually being fixed as S1 - s in O . sativa . In another lineage, the intermediate structures ( A4 - TP and TP - A6 ) carrying the new genes S1A4 ( A4 ) and S1A6 ( A6 ) arose in ancient wild rice, and the A4 - TPR-A6 three-gene structure were generated in O . barthii , probably by natural hybridization and allelic recombination; this structure further migrated into O . glaberrima as the functional S1-g allele. In hybrids between O . glaberrima and O . sativa , this gamete killer–protector system causes postzygotic reproductive isolation (PRI). b A working model for the S1 gamete killer–protector system in African-Asian rice hybrids. In the sporophytic cells (megaspore/microspore mother cells) of the hybrids, the three-protein complex, comprising TPR, A4, and A6, expressed from S1-g may produce a sterility-trigging signal. This signal is retained in the post-meiotic male and female gametes and causes the selective abortion of gametes carrying S1-s , whereas TPR in the S1-g gametes eliminates the sterility. S1-g therefore has a strong transmission advantage in the hybrids and acts as a typical ultra-selfish genetic element Full size image Despite the incomplete lineage sorting in the AA-genome Oryza species, O . meridionalis is considered to be the sister group of the other AA species [33] , [34] . Intermediate variants containing S1TP and the flanking genes S1A4 and/or S1A6 ( S1A4 - S1TP , S1TP - S1A6 , S1A4 - S1TP - S1A6 ) may therefore have appeared first in O . meridionalis , followed by the two-gene intermediate structures carrying S1TPR ( S1A4-S1TPR and S1TPR-S1A6 ) and the final functional S1A4 - S1TPR - S1A6 complex (Fig. 5a and Supplementary Fig. 13 ). These complexes probably arose during allelic recombination events in natural hybrids between ancestral species possessing the intermediate structures ( S1TPR / S1A4-S1TP , S1TPR / S1TP-S1A6 , and S1A4-S1TPR / S1TPR-S1A6 ) (Fig. 5a and Supplementary Fig. 13 ), finally generating S1A4-S1TPR-S1A6 in the O . barthii lineage. All 133 analyzed accessions of O . glaberrima were found to possess the complete S1A4-S1TPR-S1A6 structure, the same allele (Allele 2–4) was detected in O . barthii , indicating that the S1-g allele had been fixed in African rice (Fig. 5a , Supplementary Figs. 12 and 13 ). In addition, 13 accessions of O . meridionalis possessed another structure of S1A4 - S1TPR - S1A6 , where S1TPR is the primitive form of Allele 1 (Supplementary Figs. 12 and 13 ). A working model for the S1 -mediated killer–protector system Our results revealed that the three closely linked genes S1A4 , S1TPR , and S1A6 at the S1-g allele constitute a tripartite gamete killer–protector complex that acts as an ultra-selfish genetic complex generating a sterility signal via physical interaction of the three encoded proteins in the sporophytic cells. S1TPR also serves as a protector in S1-g gametophytic cells (Fig. 5b ). In O . glaberrima plants with a homozygous S1-g allele, all gametes escape abortion because S1TPR eliminates the detrimental effect induced by S1-g . The S1-s allele in O . sativa harbors only the defective S1TP gene and lacks the functional gamete killer and protector; therefore, all gametes are viable. In the interspecific hybrids, the tripartite S1A4 - S1TPR - S1A6 complex of S1 - g causes the selective abortion of gametes containing the S1-s allele, resulting in a transmission advantage for S1 - g (Fig. 5b ). To date, there are two genetic models for HS in rice [19] . The HS loci S5 , S7 , Sa , Sc , and qHMS7 fit the one-locus model [8] , [12] , [14] , [15] , [29] , while S27 / S28 , DPL1 / DPL2 , and DGS1 / DGS2 fit the two-locus model [25] , [26] , [28] . There is emerging molecular evidence to support the conclusion that the loci involved in one-locus HS systems are usually complex loci, comprising multiple adjacent and functionally related genes, as we previously reported for the Sa locus containing the adjacent genes SaF and SaM [8] . In the Sa and S5 systems, the symmetric allelic HS interactions are represented by the molecular interactions of the proteins from both alleles of the parental lines [8] , [14] ; for example, the interacting proteins in the three-component Sa complex, SaF + and SaM + , are contributed by the indica allele, while the SaM – protein is encoded by the japonica allele [8] . Similarly, in the S5 gamete-killer system, the ORF5+ protein is encoded by the indica allele, but ORF4+ is contributed by the japonica allele [14] . S1 is considered the predominant HS locus found in Oryza , because of its strong genetic effect on HS of male and female gametes in interspecific hybrid progenies. In this study, we showed that the functional African rice allele, S1-g , consists of three closely linked actively expressed genes S1A4 , S1TPR , and S1A6 ( SSP ) (Fig. 5b ). The gamete-killer function of the S1 HS system requires all the three components (S1A4, S1TPR and S1A6) only from S1-g , while the protector function depends on solely on S1-g- derived S1TPR; no component from the Asian rice allele is required for this gamete killer–protector system. The S1 gamete killer–protector system is therefore determined by the African rice allele, representing an asymmetric allelic interaction. This characteristic is distinct from the S5 and Sa systems, which are symmetric allelic interactions involving components from both divergent alleles. The S1TPR has dual roles in killer and protector function, which is distinguished from the reported killer–protector systems [14] , [15] , in which killer and protector are conferred by different factors. Thus, this S1 gamete killer–protector system expands our understanding of the single-locus BDM model. According to our transcriptome sequencing analysis, six genes in the BCAA degradation pathway were expressed at significantly lower levels in the RP- s plants than in the F 1 and NIL- g plants (Supplementary Figs. 8 – 10 ). Dysfunctional BCAA biosynthesis is known to cause the abortion of both male and female gametophyte development [35] . Therefore, we propose that the complex of the three S1-g gene products may induce excessive BCAA degradation in the F 1 and NIL- g plants, resulting in the sterility effect that affects gamete development. The S1TPR produced in S1-g -type gametes may result in adequate levels of BCAA via its peptidase function, as it resembles trypsin peptidase in animals [36] . The gametes carrying S1-s in the F 1 hybrids lacking functional S1TPR would fail to restore fertility due to their BCAA deficiency. In Asian rice cultivars ( S1-sS1-s ), the genes involved in BCAA degradation are expressed at low levels, meaning that the gametes have enough BCAA to continue their development. In addition, we reasoned that the upregulation of photosynthesis-related genes in the F 1 and NIL- g plants may be the result of a regulatory feedback loop monitoring nutrient or energy deficiency (Supplementary Figs. 8 and 10 ), which is an interesting topic for future study. The hypothesized Gondwanaland origin of the Oryza genus explains the extensive geographic distribution of the Oryza in modern species [17] , [18] , [37] . However, the current divergence times estimated from the molecular evolution between species in the Oryza genus are not in accordance with this theory [34] , [38] . These divergence times were based on sequencing analysis of the currently available species, which may cause artifacts or bias in the algorithm used due to the inability to sequence extinct ancestral species. If the Oryza genus did indeed originate in Gondwanaland, we can hypothesize that the S1 alleles in Asian rice and African rice might have originated from a common progenitor in Gondwanaland, and later evolved in parallel but independent lineages after their geographical separation (Fig. 5a ). The ancient Oryza populations located on the ancient Australian continent might have been separated from the majority of the Oryza taxa due to the breakup of Gondwanaland and subsequent continental drift, causing the S1TP allele variants (without S1A4 or S1A6 ) to pass through a genetic bottleneck before entering the O . rufipogon and O . sativa lineages in Asia. Nevertheless, other intermediate structures of S1TPR and/or S1TP variants carrying S1A4 and/or S1A6 in the ancestral Oryza species might have continued to evolve on the ancient supercontinent. The functional S1A4 - S1TPR - S1A6 structure was eventually generated in the O . barthii lineage and was further transferred into O . glaberrima and fixed on the African continent. The origin and evolution of the S1 alleles, from the intermediate (neutral) haplotypes ( S1A4-S1TPR and S1TPR-S1A6 ) to the functional ultra-selfish genetic complex, might therefore be associated with or contribute to the speciation of the related Oryza species. Polymorphism has been shown to be inevitable in the progression from allele origination to fixation at BDM loci [4] , consistent with the formation of the S1 HS allele (Supplementary Figs. 12 and 13 and Supplementary Data 1 ). Extensive sequence variations were observed in S1TPR and S1TP at the S1 locus in wild rice species (Supplementary Figs. 12 and 13 and Supplementary Data 1 ), allowing us to propose that their common ancestral sequences may be polymorphic in the Oryza species. Although the outline of the Oryza phylogeny is clear, the exact relationships among the Oryza species are elusive due to discordance between the phylogenetic trees for different genes. These issues are caused by factors such as incomplete lineage sorting [34] , [39] , [40] , meaning that the S1 alleles in Asian rice and African rice might have originated from an unknown common progenitor. The geographical distribution of polymorphisms at the S1 locus might have arisen from the long-distance dispersal of these species, which was followed by selection and fixation. Besides S1 described in this study, several other complex HS loci that are composed of two or three closely linked HS genes (such as Sa , S5 and qHMS7 ) have been identified in Oryza species [8] , [14] , [15] . These findings suggest that during speciation, generation of such complex HS loci may have advantages such as simple inheritance (as single functional genetic units having minimum recombination between the closely linked genes/alleles) and maximum genetic effect for postzygotic reproductive isolation. The functional S1-g system is predominantly fixed in O . glaberrima populations, which explains why researchers failed to identify natural hybrid-compatible (neutral) S1 alleles that could be used to break down the reproductive barrier in interspecific crosses between O . glaberrima and O . sativa . Our findings suggest that artificial hybrid-compatible S1 alleles could be created for the utilization of distant heterosis by disrupting any one of the three genes in S1-g by CRISPR/Cas9 knockout [12] , [27] , [41] . As an alternative strategy, replacing the premature stop codon in O . sativa cultivars, using base editing [42] would rescue S1TP to functional S1TPR and thereby allow gamete normal development in interspecific hybrids. Plant materials A near-isogenic line NIL- g containing S1 - g was developed using an African rice ( O . glaberrima ) line IRGC102203 as the S1 donor and an Asian rice ( O . sativa ) line IRAT216 containing S1-s as the recurrent parent (RP- s ). The genomic sequences of S1TPR , S1A4 , and S1A6 were amplified by specific primers from BAC OG-BBa0049I08, which was kindly provided by Dr. Rod A. Wing (the University of Arizona). The genomic sequences were sub-cloned into the binary vector pCAMBIA1300 using a Gibson assembly assay to generate the functional complementation constructs [43] . The target sites were fused with sgRNA expression cassettes and sub-cloned into the CRISPR/Cas9 constructs [44] for knocking out genes S1A2 – S1A6 . All functional complementation constructs and knockout plasmids were transformed into RP- s and NIL- g , using the Agrobacterium tumefaciens- mediated method. The primers used for vector construction are listed in Supplementary Table 8 . Phenotyping of pollen and spikelet fertility The plant materials were grown in Guangzhou, China during the normal growing season and in Sanya, China during the winter season. The anthers of 3–5 mature flowers from each independent flowering individual were stained with I 2 -KI solution to enable the observation and imaging of pollen fertility using a light microscope (Axio Observer D1, Carl Zeiss, Oberkochen, Germany). When the seeds ripened, the spikelet fertility was examined as the seed-setting rate in the main panicle of each individual. Histological analysis The histological analysis was performed using paraffin sectioning method [23] . Briefly, spikelets of RP- s , NIL- g , the F 1 plants from the RP- s × NIL- g and the F 1 plants from the S1A4 – S1A6 t × S1TPR t cross were fixed in FAA (1:1:18, formalin:glacial acetic acid:50% ethanol) for at least 24 h. Their ovules were then dehydrated, embedded in paraplast and cut into 8-μm longitudinal sections. The sections were stained with toluidine blue before being observed using a light microscope. Genotyping of transgenes and S1 alleles in F 2 populations The T-DNA flanking sequences of S1TPR t and S1A4 – S1A6 t were determined using hiTAIL-PCR [45] . Plants were genotyped for their T-DNA tag using PCR with the specific primer sets (Supplementary Table 8 ). In addition, the genotypes of S1 -alleles were determined by the S1 -linked In/Del marker 2170 [27] (Supplementary Table 8 ). Reverse transcription, expression and transcriptome analyses The anthers, panicles and microspores were collected from PR- s and NIL- g at different stages and their total RNA were extracted. For each sample, 2 μg of total RNA was reverse transcribed to synthesize the first-strand cDNA according to the manufacturer’s instructions (Toyobo, Osaka, Japan). The quantitative RT-PCR was conducted using gene-specific primers (Supplementary Table 8 ) with three biological replicates [46] . The data were normalized using OsActin1 as the endogenous control. The transcriptome sequencing of the anther samples was performed by GENE DENOVO Co. Ltd (Guangzhou, China). Genes with a significantly different expression level (upregulated by at least 2.82-fold or downregulated by at least 0.35 fold) in the F 1 and NIL- g plants relative to RP- s were selected for further analysis. The genes that were commonly upregulated or downregulated in the F 1 and NIL- g plants were identified and analyzed using the KEGG pathway database ( http://www.genome.jp/kegg/ ). The expression patterns of the differentially expressed genes involved in high-scoring pathways were further validated using quantitative RT-PCR. Subcellular localization and BiFC assays The coding sequences of S1TPR , S1A4 , and S1A6 were cloned into the pLYd1GFP vector carrying the GFP tag to assess their subcellular localization. They were also cloned into pVN and pVC and were fused with the N-terminal or C-erminal sequence of YFP , respectively, for the BiFC assay [47] . The plasmids were transfected into rice protoplasts followed by 15 h incubation in dark at 30 °C, after which their fluorescence was imaged using confocal microscopy (LSM 780 DUO, Carl Zeiss, Oberkochen, Germany). In vitro protein pull-down assay The pull-down assays were conducted according to the manufacturer’s instructions (New England Biolabs, MA, USA). Briefly, the S1A4 protein was fused to an MBP-tag as the bait, while the S1A6 or S1TPR proteins were fused with a GST-tag as the prey. The MBP-S1A4, GST-S1A6, or GST-S1TPR proteins were expressed in Escherichia coli Rosetta (DE3). The cells containing these recombinant proteins were harvested in phosphate-buffered saline (pH 7.4) and then were ruptured by sonication. The lysates containing MBP-S1A4 were pulled down using amylose resin and mixed with lysates containing GST-S1A6 or GST-S1TPR. The proteins were pulled down and detected using western blotting with anti-MBP (TransGen Biotech, Beijing, China, #HT701, 1:5000 dilution) and anti-GST antibodies (TransGen Biotech, Beijing, China, #HT601, 1:5000 dilution), respectively. Uncropped blots are presented in the Source Data file. Phylogenetic and evolutionary analysis of the S1 locus To determine the orthologs of S1A4 , S1A6 , and S1TPR , their nucleotide sequences were used as templates in a BLAST search of the Poaceae family in the GenBank database ( https://www.ncbi.nlm.nih.gov/ ). The sequences of the putative orthologs were downloaded and used for the phylogenetic study. The phylogenetic tree was constructed using the maximum likelihood method via MEGA7 ( www.megasoftware.net/ ), with 1,000 bootstrap replications. To trace the ancestral S1TPR and S1TP sequences, seven non-synonymous SNPs were analyzed in two accessions of S . italica and 458 rice accessions. For the bioinformatics analysis, the publicly available sequences from the OMAP project [48] , [49] , the wild rice genome project [50] , the 3000 rice genomes project [51] and the African wild rice genome [52] were downloaded from NCBI. The short reads were aligned to the genomic sequences of the S1-g and S1-s alleles using Burrows-Wheeler Aligner [53] . The depth of coverage and the SNPs were detected using the SAMtools package [54] . To determine the presence of S1A4 and S1A6 , coverage was calculated based on their depth at each nucleotide position with a Python program. Primer sets covering the genomic region of S1TPR , S1TP , S1A4 , and S1A6 were designed to amplify the target region for the validation of the sequences in several collected accessions of wild and cultivated rice species to trace the divergence of the S1 locus.